Chemical and genetic validation of thiamine utilization as an antimalarial drug target Thiamine is metabolized into an essential cofactor for several enzymes. Here we show that oxythiamine, a thiamine analog, inhibits proliferation of the malaria parasite Plasmodium falciparum in vitro via a thiamine-related pathway and significantly reduces parasite growth in a mouse malaria model. Overexpression of thiamine pyrophosphokinase (the enzyme that converts thiamine into its active form, thiamine pyrophosphate) hypersensitizes parasites to oxythiamine by up to 1,700-fold, consistent with oxythiamine being a substrate for thiamine pyrophosphokinase and its conversion into an antimetabolite. We show that parasites overexpressing the thiamine pyrophosphate-dependent enzymes oxoglutarate dehydrogenase and pyruvate dehydrogenase are up to 15-fold more resistant to oxythiamine, consistent with the antimetabolite inactivating thiamine pyrophosphate-dependent enzymes. Our studies therefore validate thiamine utilization as an antimalarial drug target and demonstrate that a single antimalarial can simultaneously target several enzymes located within distinct organelles. During its intraerythrocytic cycle, the human malaria parasite Plasmodium falciparum requires several extracellular nutrients to support its proliferation. Until recently, an extracellular supply of thiamine (vitamin B 1 ) was not believed to be essential to the parasite, because (i) previous data were consistent with pantothenate (vitamin B 5 ) being the only extracellular vitamin required by the parasite [1] , [2] and (ii) genes coding for thiamine biosynthesis enzymes had been identified in the parasite’s genome [3] , [4] and their functionality analysed using a heterologous approach [5] . Recent work, however, demonstrated that depletion of thiamine from erythrocytes is detrimental to parasite growth. Therefore, although the parasite is capable of synthesizing thiamine, its capacity to do so appears to be insufficient to meet its requirements [6] . The parasite’s thiamine biosynthesis pathway has been suggested to be a target for novel and much-needed antimalarials, either by direct inhibition of the enzymes or by channelling prodrugs into this parasite specific pathway [7] . However, interfering with the thiamine biosynthesis enzymes as an antimalarial strategy is promising only if the parasite is unable to source sufficient quantities of the vitamin extracellularly. The uptake and/or utilization of thiamine, therefore, represent more suitable targets, as inhibition of these processes should inhibit parasite proliferation. Once synthesized (or taken up) by the parasite, thiamine is pyrophosphorylated by the enzyme thiamine pyrophosphokinase ( Pf TPK) to generate thiamine pyrophosphate (TPP) [8] , the active form of thiamine [9] . TPP is central to the activity of several enzymes [10] , [11] , particularly those involved in the metabolism of glucose. In P. falciparum , a number of enzyme activities are predicted to depend on TPP, including the E1 subunits of pyruvate dehydrogenase (PDH) and 2-oxoglutarate dehydrogenase (OxoDH), 3-methyl-2-oxobutanoate dehydrogenase, 1-deoxy- D -xylose phosphate synthase and transketolase [3] , [7] . Only three of these enzymes have been investigated so far in P. falciparum : (i) the PDH complex in the apicoplast, an algae-derived organelle in which fatty acid biosynthesis occurs [12] , (ii) the OxoDH complex in the mitochondrion [13] and (iii) transketolase, the key enzyme of the non-oxidative arm of the pentose phosphate pathway [14] . Although these enzymes have been proposed to be potential drug targets, their essentiality to the intraerythrocytic growth of P. falciparum is still unclear. In fact, in a recent study using Plasmodium yoelii (a mouse malaria species), PDH has been shown to be essential only for the parasite’s progression from the liver stage [15] . It remains to be seen whether this is also the case for P. falciparum and whether PDH (or any of the other TPP-dependent enzymes) might serve as an antimalarial drug target. In this study, we have used the thiamine analog, oxythiamine, genetically modified P. falciparum parasites and heterologously expressed P. falciparum enzymes to investigate whether thiamine utilization is a viable antimalarial drug target. We show that oxythiamine not only inhibits parasite growth in vitro but also in vivo in a mouse model of malaria. We go on to show that oxythiamine competes with thiamine as a substrate for TPK and that the resulting antimetabolite, oxythiamine pyrophosphate (OxPP), interacts with the parasite TPP-dependent enzymes PDH and OxoDH. Furthermore, we provide evidence that the parasite PDH and OxoDH E1 subunits are able to accept both pyruvate and oxoglutarate as substrates, raising the possibility that each enzyme is capable of compensating the loss of activity of the other. Inhibition of P. falciparum growth in vitro by oxythiamine The thiamine analog oxythiamine ( Fig. 1a ) inhibited the in vitro proliferation of the 3D7 strain of P. falciparum with an IC 50 value of 5.2±0.3 mM (mean±s.e.m. ; n =6). In the absence of extracellular thiamine (that is, in thiamine-free culture medium), a significant increase in parasite sensitivity to oxythiamine was observed ( Fig. 1b ), resulting in a 450-fold decrease in the IC 50 value (11±4 μM; mean±s.e.m. ; n =6; P =0.002, Mann–Whitney U -test). Increasing the thiamine concentration in the thiamine-replete culture medium by 100-fold (to 296 μM), however, had no significant effect on the antiplasmodial potency of oxythiamine (IC 50 =5.5±0.5 mM; mean±s.e.m. ; n =6; P =0.81, Mann–Whitney U -test; Fig. 1b ). We also tested the antiplasmodial activity of oxythiamine in the presence of 50 nM thiamine (the upper limit of the physiological plasma thiamine concentration [16] ). We found that at this extracellular thiamine concentration, oxythiamine inhibited parasite growth with an IC 50 of 23±3 μM (mean±s.e.m. ; n =3; Fig. 1b ). 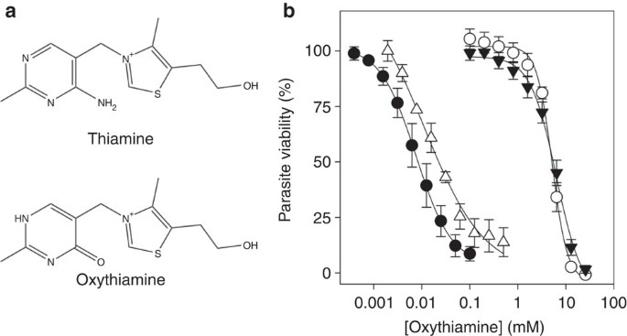Figure 1: Oxythiamine structure andin vitroantiplasmodial activity. (a) Chemical structures of thiamine and oxythiamine. (b)In vitroantiplasmodial activity of oxythiamine againstP. falciparum(strain 3D7) in thiamine-free RPMI-1640 medium (filled circles), and in the presence of 50 nM (open triangles), 2.96 μM (open circles) or 296 μM thiamine (filled triangles). The data are averaged from three (open triangles) or six (all the others) independent experiments, each performed in duplicate and are shown ±s.e.m. Where not shown, error bars are smaller than the symbols. Figure 1: Oxythiamine structure and in vitro antiplasmodial activity. ( a ) Chemical structures of thiamine and oxythiamine. ( b ) In vitro antiplasmodial activity of oxythiamine against P. falciparum (strain 3D7) in thiamine-free RPMI-1640 medium (filled circles), and in the presence of 50 nM (open triangles), 2.96 μM (open circles) or 296 μM thiamine (filled triangles). The data are averaged from three (open triangles) or six (all the others) independent experiments, each performed in duplicate and are shown ±s.e.m. Where not shown, error bars are smaller than the symbols. Full size image Antiplasmodial activity of oxythiamine in vivo To investigate whether oxythiamine also possesses antiplasmodial activity in vivo , we administered oxythiamine (400 mg kg −1 per day for 3 days) orally to mice infected with Plasmodium vinckei vinckei and monitored the parasitemia and survival of the mice over 8 days. The parasitemia on day 5 post infection of oxythiamine-treated mice was significantly lower, by almost sixfold, than that of vehicle (water)-treated mice ( n =8; P<< 0.001, Student’s t -test; Fig. 2a ). The survival time of oxythiamine-treated mice, relative to vehicle-treated mice, was also prolonged ( P<< 0.001, Student’s t -test; Fig. 2b ). As shown in Fig. 2c , the average body weight of mice in the control group did not change during the course of the experiment. However, body weight declined progressively with each daily dose of oxythiamine. After three doses, the average body weight of the mice had decreased by 13% ( P =0.0002, Student’s t -test). Following cessation of oxythiamine administration, all but one of the mice regained weight, such that 3 days after the administration of the final dose, the average weight of the mice was statistically indistinguishable from their starting weight ( P =0.16, Student’s t -test). The one mouse that continued to lose weight had a detectable parasitemia and was euthanized. 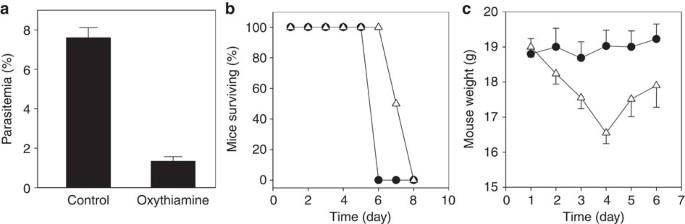Figure 2:In vivoantimalarial activity of oxythiamine. (a) Average parasitemia at day 5 post infection/start of treatment inP. vinckei vinckei-infected mice treated orally with vehicle (water) control and oxythiamine (400 mg kg−1per day for 3 days). Error bars represent s.e.m. (n=7–8). (b) Survival time of mice following treatment with vehicle control (filled circles) and oxythiamine (open triangles; 400 mg kg−1per day for 3 days) starting on the day of infection. (c) Average weight of mice treated orally with water (vehicle control; filled circles) and oxythiamine (open triangles). Error bars represent s.e.m. (n=7–8). For clarity, only positive or negative error bars are shown. Figure 2: In vivo antimalarial activity of oxythiamine. ( a ) Average parasitemia at day 5 post infection/start of treatment in P. vinckei vinckei -infected mice treated orally with vehicle (water) control and oxythiamine (400 mg kg −1 per day for 3 days). Error bars represent s.e.m. ( n =7–8). ( b ) Survival time of mice following treatment with vehicle control (filled circles) and oxythiamine (open triangles; 400 mg kg −1 per day for 3 days) starting on the day of infection. ( c ) Average weight of mice treated orally with water (vehicle control; filled circles) and oxythiamine (open triangles). Error bars represent s.e.m. ( n =7–8). For clarity, only positive or negative error bars are shown. Full size image Oxythiamine interacts with Pf TPK One potential target of oxythiamine in the parasite is Pf TPK. Overexpression of Pf TPK would therefore be expected to render the parasites resistant to oxythiamine. To investigate this possibility, we generated a parasite line expressing extra copies of Pf TPK (referred to as 3D7-TPK + ). The episomally expressed copies of Pf TPK contained a C-terminal streptavidin (strep) tag to allow confirmation of protein expression. As demonstrated in Fig. 3a , anti-strep antibodies readily detected the tagged version of Pf TPK, which is absent in 3D7 parasites transfected with a mock plasmid (3D7-Mock [17] ). As expected, anti- Pf TPK antibodies detected two bands in western blots of 3D7-TPK + (consistent with the endogenous (smaller band) and episomally expressed tagged versions of Pf TPK) and only a single band in those prepared from wild-type 3D7 parasites ( Fig. 3a ). The growth rate of 3D7-TPK + was comparable to that of 3D7-Mock ( Supplementary Fig. S1 ). The sensitivity of 3D7-TPK + to oxythiamine was compared with that of 3D7-Mock in thiamine-replete and thiamine-free culture medium. 3D7-TPK + was 1,700-fold ( Fig. 3b ) and 70-fold ( Fig. 3c ) more sensitive than 3D7-Mock to oxythiamine in thiamine-replete and thiamine-free culture medium, respectively (IC 50 =4.6±1.4 μM; mean±s.e.m. ; n =5; P =0.00046, Mann–Whitney U -test, and IC 50 =0.25±0.05 μM; mean±s.e.m. ; n =5; P =0.0016, Mann–Whitney U -test, in thiamine-replete and thiamine-free culture medium, respectively). As expected, the sensitivity of the 3D7 and 3D7-Mock parasite lines to oxythiamine was similar in both culture media (data not shown). 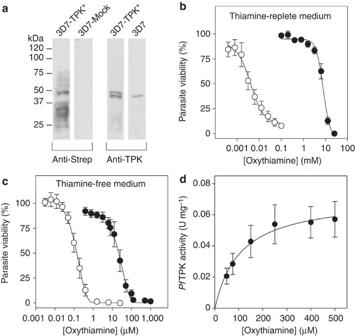Figure 3: Analysis of 3D7-TPK+parasites andin vitrophosphorylation of oxythiamine. (a) Western blot analysis of 3D7-TPK+using monoclonal anti-strep (first two lanes) and anti-TPK antibodies (last two lanes). Wild-type 3D7 parasites and 3D7-Mock are used as controls. (b) Antiplasmodial activity of oxythiamine againstP. falciparum3D7-Mock (filled circles) and 3D7-TPK+(open circles) parasite lines in thiamine-replete culture medium. (c) Antiplasmodial activity of oxythiamine againstP. falciparum3D7-Mock (filled circles) and 3D7-TPK+(open circles) parasite lines in thiamine-free culture medium. The data are averaged from at least three independent experiments, each performed in duplicate and are shown ±s.e.m. Where not shown, error bars are smaller than the symbols. (d) Michaelis–Menten analysis of oxythiamine pyrophosphorylation using heterologously expressed and purifiedPfTPK (KMof 145±31 μM). The data were analysed with SigmaPlot and are averaged from four independent experiments, each carried out in duplicate and are shown ±s.e.m. Figure 3: Analysis of 3D7-TPK + parasites and in vitro phosphorylation of oxythiamine. ( a ) Western blot analysis of 3D7-TPK + using monoclonal anti-strep (first two lanes) and anti-TPK antibodies (last two lanes). Wild-type 3D7 parasites and 3D7-Mock are used as controls. ( b ) Antiplasmodial activity of oxythiamine against P. falciparum 3D7-Mock (filled circles) and 3D7-TPK + (open circles) parasite lines in thiamine-replete culture medium. ( c ) Antiplasmodial activity of oxythiamine against P. falciparum 3D7-Mock (filled circles) and 3D7-TPK + (open circles) parasite lines in thiamine-free culture medium. The data are averaged from at least three independent experiments, each performed in duplicate and are shown ±s.e.m. Where not shown, error bars are smaller than the symbols. ( d ) Michaelis–Menten analysis of oxythiamine pyrophosphorylation using heterologously expressed and purified Pf TPK ( K M of 145±31 μM). The data were analysed with SigmaPlot and are averaged from four independent experiments, each carried out in duplicate and are shown ±s.e.m. Full size image The increased sensitivity of 3D7-TPK + to oxythiamine is not consistent with Pf TPK being the target of oxythiamine. It is consistent, however, with oxythiamine being a substrate for Pf TPK, and with the overexpressed Pf TPK generating a higher concentration of a toxic oxythiamine metabolite within the parasite. We therefore tested whether oxythiamine is a substrate for heterologously expressed Pf TPK. Oxythiamine was indeed metabolized by Pf TPK with a K M value of 145±31 μM and a specific activity of 79±14 nmol min −1 mg −1 (mean±s.e.m. ; n =4; Fig. 3d ). Downstream effect on TPP-dependent enzymes In light of the fact that Pf TPK accepts oxythiamine as a substrate, presumably generating OxPP, we explored the hypothesis that the mechanism of action of oxythiamine is via the generation of toxic OxPP that interacts with TPP-dependent enzymes, rendering them non-functional. To test this hypothesis, we generated two additional transgenic parasite lines expressing extra copies of either the TPP-binding subunit of the P. falciparum PDH E1-α (3D7-PDH + ) or the E1 subunit of the P. falciparum OxoDH (3D7-OxoDH + ). To confirm their expression within the parasite, the constructs were strep-tagged and visualized as single bands of the expected size on western blots using a monoclonal anti-strep antibody ( Fig. 4a ). The growth rates of 3D7-OxoDH + and 3D7-PDH + were similar to that of 3D7-Mock and 3D7-TPK + ( Supplementary Fig. S1 ). 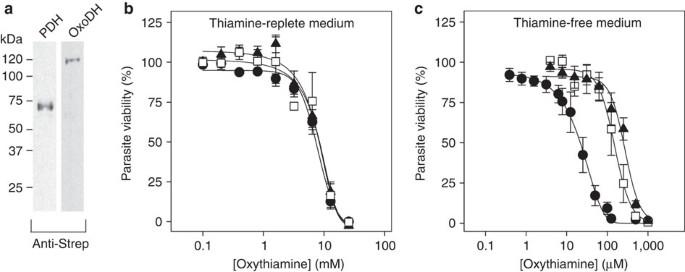Figure 4: Analysis of 3D7-PDH+and 3D7-OxoDH+transgenic parasite lines. (a) Western blot analysis of transgenic parasites using monoclonal anti-strep antibodies. (b) Antiplasmodial activity of oxythiamine againstP. falciparum3D7-Mock (filled circles), 3D7-OxoDH+(open squares) and 3D7-PDH+(filled triangles) lines in thiamine-replete culture medium. (c) Antiplasmodial activity of oxythiamine againstP. falciparum3D7-Mock (filled circles), 3D7-OxoDH+(open squares) and 3D7-PDH+(filled triangles) lines in thiamine-free culture medium. The data are averaged from at least three independent experiments, each performed in duplicate and showed ±s.e.m. Where not shown, error bars are smaller than the symbols. Figure 4: Analysis of 3D7-PDH + and 3D7-OxoDH + transgenic parasite lines. ( a ) Western blot analysis of transgenic parasites using monoclonal anti-strep antibodies. ( b ) Antiplasmodial activity of oxythiamine against P. falciparum 3D7-Mock (filled circles), 3D7-OxoDH + (open squares) and 3D7-PDH + (filled triangles) lines in thiamine-replete culture medium. ( c ) Antiplasmodial activity of oxythiamine against P. falciparum 3D7-Mock (filled circles), 3D7-OxoDH + (open squares) and 3D7-PDH + (filled triangles) lines in thiamine-free culture medium. The data are averaged from at least three independent experiments, each performed in duplicate and showed ±s.e.m. Where not shown, error bars are smaller than the symbols. Full size image If either Pf OxoDH or Pf PDH is essential for parasite survival during its intraerythrocytic stage, and if the antiplasmodial activity of oxythiamine is via the generation of OxPP that inactivates one or both of these enzymes, overexpression of the inhibited enzymes should render the parasite relatively resistant to oxythiamine compared with wild-type parasites. We therefore explored the sensitivity of 3D7-OxoDH + and 3D7-PDH + to oxythiamine in thiamine-free and thiamine-replete culture medium. The sensitivity of 3D7-PDH + and 3D7-OxoDH + to oxythiamine in thiamine-replete culture medium was indifferent to that of 3D7-Mock (IC 50 =8.1±0.9 mM; n =7 and 8.4±1.4 mM; n =4, respectively; mean±s.e.m. ; P >0.75, Mann–Whitney U -test; Fig. 4b ). On the other hand, in thiamine-free culture medium, 3D7-OxoDH + and 3D7-PDH + were 15-fold (IC 50 =263±39 μM; mean±s.e.m. ; n =3; P =0.012, Mann–Whitney U -test) and 9-fold (IC 50 =158±42 μM; mean±s.e.m. ; n =4; P =0.004, Mann–Whitney U -test) more resistant to oxythiamine, respectively ( Fig. 4c ). To exclude the possibility that the altered oxythiamine sensitivity observed in the 3D7-PDH + , 3D7-OxoDH + and 3D7-TPK + transgenic parasites ( Figs 3b,c and 4c ) is due to off-target effects generated during the drug-selection process, we tested their sensitivity to the antimalarial chloroquine and found that it was unaltered ( Supplementary Fig. S2 ). Furthermore, to confirm overexpression of the target genes, we used quantitative PCR to compare the mRNA levels of Pf PDH, Pf OxoDH and Pf TPK in the transgenic parasites relative to their mRNA levels in 3D7-Mock parasites ( Fig. 5 ). We found significantly higher levels of mRNA for all three genes in the corresponding transgenic parasite line (11±2-, 4.4±0.4- and 8.0±0.6-fold increases for Pf PDH, Pf OxoDH and Pf TPK, respectively; mean±s.e.m. ; n =4–10; P <0.001 in each case, analysis of variance+Dunnett’s test). 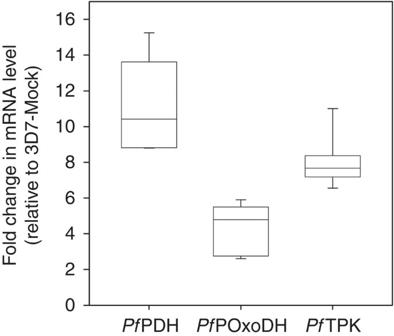Figure 5: mRNA expression in transgenic parasite lines. The data are normalized to aldolase, and the fold change inPfPDH,PfOxoDH andPfTPK mRNA expression is shown relative to the levels observed in 3D7-Mock parasites. The box indicates the 25–75 percentiles, the error bars show the range and the middle line represents the median. The data were generated from 4–10 independent experiments. Figure 5: mRNA expression in transgenic parasite lines. The data are normalized to aldolase, and the fold change in Pf PDH, Pf OxoDH and Pf TPK mRNA expression is shown relative to the levels observed in 3D7-Mock parasites. The box indicates the 25–75 percentiles, the error bars show the range and the middle line represents the median. The data were generated from 4–10 independent experiments. Full size image OxPP binds to Pf PDH and Pf OxoDH in situ The data showing that Pf TPK is able to metabolize oxythiamine in vitro ( Fig. 3d ) and that parasites overexpressing TPP-dependent enzymes are resistant to oxythiamine ( Fig. 4c ) are consistent with the parasite converting oxythiamine to OxPP and with OxPP inactivating one or more TPP-dependent enzymes. To investigate this, we used high-performance liquid chromatography (HPLC) to detect OxPP generated by the parasite from oxythiamine in situ and which had been immobilized from parasite-purified Pf PDH and Pf OxoDH. Thiamine, oxythiamine, TPP and OxPP had distinct retention times of 0.875, 0.695, 0.605 and 0.432 min, respectively, and were easily detectable ( Fig. 6 ). We then treated erythrocytes infected with 3D7-PDH + and 3D7-OxoDH + trophozoites with the IC 50 concentration of oxythiamine (5.2 mM) in the presence of thiamine (2.96 μM) or the IC 50 concentration of oxythiamine (11 μM) in the absence of thiamine ( Fig. 1 ) for 5 h, and purified the strep-tagged Pf PDH E1 and Pf OxoDH E1 subunits via affinity chromatography from the corresponding transgenic parasites. Control parasites incubated in the presence of thiamine, but in the absence of oxythiamine, were also analysed. Cofactors that co-eluted with the purified proteins were then detected using HPLC. A single major metabolite was co-purified with both proteins ( Fig. 6 ) under all experimental conditions. As expected, in oxythiamine-free control samples ( Fig. 6a ) the cofactor from both Pf PDH and Pf OxoDH had a retention time of 0.609±0.003 min (mean±range/2), consistent with the cofactor being TPP. In oxythiamine-treated samples, the major metabolite had a retention time of 0.433±0.002 min (mean±s.e.m.) for both Pf PDH E1 ( Fig. 6b ) and Pf OxoDH E1 ( Fig. 6e ) subunits, consistent with the cofactor being OxPP. To confirm that the peak derived from oxythiamine-treated parasites was not TPP, samples were ‘spiked’ with TPP and re-analysed by HPLC ( Fig. 6b , dashed lines). The cofactor bound to the target proteins in oxythiamine-treated samples is clearly distinct from the natural cofactor TPP (asterisks in Fig. 6 ). Our data, therefore, are consistent with the parasite synthesizing OxPP in situ and with OxPP binding to TPP-dependent enzymes. 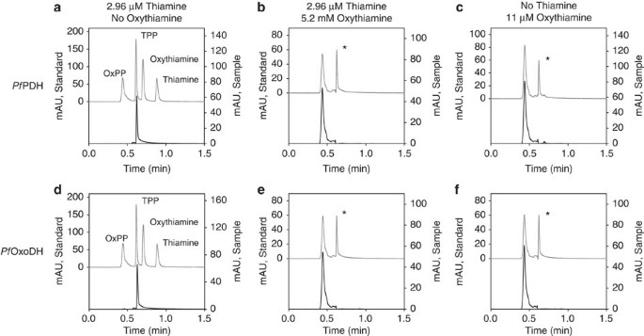Figure 6: Detection of TPP and OxPP bound toPfPDH andPfOxoDH. HPLC analysis showing the major metabolite detected from strep-tagged affinity-purifiedPfPDH from 3D7-PDH+parasites (a–c) andPfOxoDH from 3D7-OxoDH+parasites (d–f) incubated in normal RPMI-1640 (a,d), normal RPMI-1640 in the presence of 5.2 mM oxythiamine (b,e) and thiamine-free RPMI-1640 in the presence of 11 μM oxythiamine (c,f). Inbandc, the dashed lines in the background show the separation of the standards (OxPP, TPP, oxythiamine and thiamine) to enable the identification of the metabolite. The dashed lines inb,c,eandfrepresent an identical sample as that shown by the solid line, but which had been ‘spiked’ with 1 μM TPP (peak indicated by the asterisk) to illustrate that the cofactor bound to the target protein when the parasites had been treated with IC50concentrations of oxythiamine is distinct from TPP. The traces are representative of those obtained in two independent affinity-purification experiments. Figure 6: Detection of TPP and OxPP bound to Pf PDH and Pf OxoDH. HPLC analysis showing the major metabolite detected from strep-tagged affinity-purified Pf PDH from 3D7-PDH + parasites ( a – c ) and Pf OxoDH from 3D7-OxoDH + parasites ( d – f ) incubated in normal RPMI-1640 ( a , d ), normal RPMI-1640 in the presence of 5.2 mM oxythiamine ( b , e ) and thiamine-free RPMI-1640 in the presence of 11 μM oxythiamine ( c , f ). In b and c , the dashed lines in the background show the separation of the standards (OxPP, TPP, oxythiamine and thiamine) to enable the identification of the metabolite. The dashed lines in b , c , e and f represent an identical sample as that shown by the solid line, but which had been ‘spiked’ with 1 μM TPP (peak indicated by the asterisk) to illustrate that the cofactor bound to the target protein when the parasites had been treated with IC 50 concentrations of oxythiamine is distinct from TPP. The traces are representative of those obtained in two independent affinity-purification experiments. Full size image Activity and localization of Pf PDH and Pf OxoDH If one considers the relative resistance to oxythiamine of the 3D7-PDH + and 3D7-OxoDH + parasite lines (when compared with 3D7-Mock) in isolation, it is reasonable to conclude that Pf PDH and Pf OxoDH are essential for parasite viability and that they are the target of oxythiamine. If considered collectively, however, it is unclear why the overexpression of Pf OxoDH should render the parasites resistant to oxythiamine if Pf PDH is the target for the antiplasmodial activity of oxythiamine. The converse is, of course, also true; if Pf OxoDH is the target, how does Pf PDH overexpression convey oxythiamine resistance to the parasites? We considered two possible explanations for this observation. The first is that both enzymes compete for the antimetabolite (OxPP). Overexpression of either enzyme would, therefore, reduce the effective concentration of OxPP within the parasite and allow the other TPP-dependent enzyme to bind to TPP and function normally. The second is that Pf PDH and Pf OxoDH are able to compensate for each other’s activity. For the second explanation to be true, Pf PDH and Pf OxoDH must accept both pyruvate and oxoglutarate as substrates, and the enzymes need to be located at the same site(s) as both substrates. To determine whether Pf PDH and Pf OxoDH are able to accept each other’s normal substrates, the activity of the recombinantly expressed E1 subunits of Pf OxoDH and Pf PDH (α and β, co-purified) was analysed biochemically. Both subunits are able to accept pyruvate and oxoglutarate as demonstrated by their similar specific activities for both substrates ( Table 1 ). Table 1 Activity profile of the recombinant E1 subunits of Pf PDH and Pf OxoDH Full size table To confirm their location within the parasite, parasites expressing green fluorescent protein (GFP)-tagged versions of the first 100 amino acids of the N terminus of each enzyme subunit were generated. The expression of the GFP chimeras in the parasite was confirmed by western blot analysis using anti-GFP antibodies ( Fig. 7a ). As described previously [12] , the E1-α subunit of Pf PDH localizes to a discrete organelle adjacent to the mitochondrion and distinct from the nucleus, consistent with an apicoplast localization ( Fig. 7b ; top panel). The truncated E1 subunit of Pf OxoDH, which has been predicted to have a mitochondrial localization [13] , colocalizes with MitoTracker when fused to GFP ( Fig. 7b ; bottom panel), consistent with a mitochondrial localization. Although the localization was as predicted, it should be noted that the tagged proteins were expressed under a non-authentic promotor, and this may influence the localization of the protein [18] . 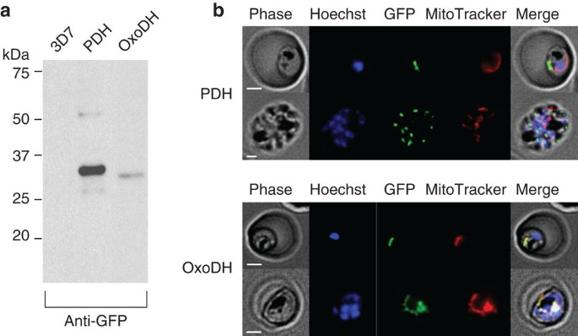Figure 7: Localization ofPfPDH andPfOxoDH within erythrocytes infected with 3D7 parasites. (a) Western blot analysis of transgenic parasites expressing GFP-tagged leader sequences ofPfPDH andPfOxoDH using monoclonal anti-GFP antibody. Wild-type 3D7 parasites are included as a control. (b) Localization ofPfPDH (top panel) andPfOxoDH (bottom panel) in transgenic parasites. The left column shows phase contrast images, followed by fluorescence images of a nuclear dye (Hoechst; blue), GFP-tagged leader sequences of the target enzymes (green), a mitochondrial dye (MitoTracker; red) and all four images merged together (right column). Scale bars, 2 μm. Figure 7: Localization of Pf PDH and Pf OxoDH within erythrocytes infected with 3D7 parasites. ( a ) Western blot analysis of transgenic parasites expressing GFP-tagged leader sequences of Pf PDH and Pf OxoDH using monoclonal anti-GFP antibody. Wild-type 3D7 parasites are included as a control. ( b ) Localization of Pf PDH (top panel) and Pf OxoDH (bottom panel) in transgenic parasites. The left column shows phase contrast images, followed by fluorescence images of a nuclear dye (Hoechst; blue), GFP-tagged leader sequences of the target enzymes (green), a mitochondrial dye (MitoTracker; red) and all four images merged together (right column). Scale bars, 2 μm. Full size image Oxythiamine has been previously shown to inhibit the in vitro growth of P. falciparum [19] , although investigations into its mechanism of action have not been carried out. Studies in yeast showed that oxythiamine reduces the uptake of thiamine by 45% (ref. 20 ) and inhibits TPP-dependent enzymes [21] . Furthermore, oxythiamine inhibits cancer cell growth by acting as a thiamine antagonist and an inhibitor of transketolase [22] . We therefore investigated whether oxythiamine inhibits P. falciparum growth by interfering with the parasite’s thiamine-utilization pathway and whether it is active in vivo . The antiplasmodial activity of oxythiamine increases in response to the extracellular thiamine concentration being reduced ( Fig. 1b ), consistent with oxythiamine interfering with the uptake and/or metabolism of thiamine in a competitive manner. In the presence of 2.96 μM thiamine, the antiplasmodial activity of oxythiamine is poor (IC 50 =5.2 mM), but in the presence of 50 nM thiamine, the upper limit of thiamine in human serum [16] , the antiplasmodial activity of oxythiamine is substantially higher, with an IC 50 of 23 μM. Increasing the extracellular thiamine concentration by 100-fold (to 296 μM) had no effect on the antiplasmodial activity of oxythiamine ( Fig. 1b ). Although it is unclear why this would be the case, one possibility is that at high concentrations, oxythiamine kills the parasite via an effect that is unrelated to thiamine utilization. Another possibility is that one or more parasite thiamine-utilization steps become saturated at high thiamine concentrations. Under these conditions, increasing the extracellular thiamine concentration further has no effect on the antiplasmodial activity of oxythiamine. Oxythiamine (400 mg kg −1 per day for 3 days) was effective at reducing the parasite burden of P. vinckei vinckei -infected mice by more than 80% ( Fig. 2a ) and increasing the survival of the mice (albeit marginally; Fig. 2b ). However, the reduction in mouse body weight ( Fig. 2c ), which we ascribe to oxythiamine-induced toxicity, is obviously undesirable, but it was also unexpected, given the results of earlier studies investigating the anti-tumour effect of oxythiamine in mice [23] , [24] . Raïs et al . [24] administered doses as high as 500 mg kg −1 per day for 4 days and lower doses of 300 mg kg −1 per day for 14 days without observing toxicity. A more recent study [25] using similar oxythiamine doses to Raïs et al . [24] , but administering the drug orally for a period of up to 5 weeks, also reported no toxicity. The discrepancy between our study and previous reports on the lack of oxythiamine toxicity [23] , [24] , [25] is unclear. It is worth noting that the high dose of oral oxythiamine required in this and previous studies may be due to a concomitant low plasma concentrations of oxythiamine, as has been previously shown to be the case for orally administered thiamine in humans [26] . Therefore, although oxythiamine is unlikely to be developed as an antimalarial in its own right, we propose that it can serve as a starting point from which to design antimalarials targeting this pathway. Another factor to consider in developing antimalarials that target the parasite’s thiamine-utilization pathway is the reported association between P. falciparum malaria and thiamine deficiency [27] , [28] . The reason for this association is unclear, but may be related to the increase in the basal metabolic rate (and hence thiamine utilization) because of the febrile nature of the illness [28] . The reduced thiamine concentrations in these individuals would be predicted to enhance the antiplasmodial activity of inhibitors that act competitively with thiamine (such as oxythiamine), but such inhibitors may also exacerbate the host’s thiamine deficiency. It is therefore important that the compounds specifically target the parasite. To investigate the mode of action of oxythiamine, we overexpressed enzymes ( Fig. 5 ) involved in the metabolism of thiamine. Parasites overexpressing Pf TPK became hypersensitive to oxythiamine ( Fig. 3b ). At least one earlier study [29] has shown increased drug sensitivity as a result of targeted overexpression of a parasite protein (involved in vitamin B 6 metabolism), but this increased sensitivity was subtle when compared with that observed here. The increased oxythiamine sensitivity of 3D7- Pf TPK + parasites, together with our demonstration that oxythiamine is a substrate of Pf TPK ( Fig. 3d ) with an affinity that is approximately only twofold lower than that of thiamine [8] , are consistent with the increased sensitivity of 3D7- Pf TPK + to oxythiamine being due to an increased generation of toxic OxPP via the action of Pf TPK (see Fig. 8 for schematic representation). 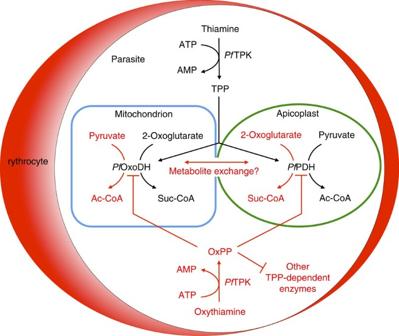Figure 8:P. falciparumthiamine utilization and mechanism of action of oxythiamine. Thiamine is metabolized to its active form, TPP, byPfTPK in an ATP-dependent manner. TPP is essential as a cofactor for the enzymesPfOxoDH in the mitochondrion andPfPDH in apicoplast. We show that the thiamine analog, oxythiamine, is metabolized byPfTPK, and the resulting metabolite, OxPP, likely inhibits the activity ofPfPDH,PfOxoDH and other TPP-dependent enzymes. The pathways shown in black represent established or previously suggested pathways, whereas the pathways in red illustrate mechanisms identified in this study or that would need to be present in order for one of the models proposed in this study to hold. Figure 8: P. falciparum thiamine utilization and mechanism of action of oxythiamine. Thiamine is metabolized to its active form, TPP, by Pf TPK in an ATP-dependent manner. TPP is essential as a cofactor for the enzymes Pf OxoDH in the mitochondrion and Pf PDH in apicoplast. We show that the thiamine analog, oxythiamine, is metabolized by Pf TPK, and the resulting metabolite, OxPP, likely inhibits the activity of Pf PDH, Pf OxoDH and other TPP-dependent enzymes. The pathways shown in black represent established or previously suggested pathways, whereas the pathways in red illustrate mechanisms identified in this study or that would need to be present in order for one of the models proposed in this study to hold. Full size image Previous P. falciparum studies have shown that overexpression of an endogenous protein can result in resistance to drugs that inhibit the overexpressed protein. Typically, these studies [30] , [31] showed relatively modest increases (2–3-fold) in IC 50 values. Our demonstration that parasites overexpressing the thiamine-binding subunits of Pf PDH or Pf OxoDH are 9- and 15-fold, respectively, more resistant to oxythiamine in thiamine-free medium ( Fig. 4c ), therefore, represents considerably larger alterations to drug sensitivity. These observations are consistent with oxythiamine being an antimetabolite. In thiamine-replete culture medium, the oxythiamine sensitivity of parasites overexpressing Pf OxoDH or Pf PDH is unchanged ( Fig. 4b ). This is not surprising, because under these conditions the parasite’s sensitivity to oxythiamine is not affected by higher extracellular thiamine concentrations ( Fig. 1b ). The fact that increased resistance to oxythiamine is observed only in thiamine-free medium is consistent with the activity being due to a thiamine-related effect, rather than a general drug-resistance phenotype. The demonstration that OxPP is synthesized by the parasite from oxythiamine and that OxPP binds to Pf OxoDH and Pf PDH in situ ( Fig. 6 ) is consistent with OxPP binding (as an unnatural cofactor) to TPP-dependent enzymes and rendering them non-functional, thereby killing the parasite ( Fig. 8 ). A similar hypothesis has been put forward for the mode of action of oxythiamine against Saccharomyces cerevisiae [21] . The P. falciparum transketolase (another TPP-utilizing enzyme) has recently been shown in in vitro studies to bind to, and be inactivated by, OxPP [32] , providing additional support for our model. It is likely that additional P. falciparum TPP-dependent enzymes are also targeted by OxPP, but this remains to be investigated. Unlike eukaryotic cells where PDH is located within mitochondria, in P. falciparum PDH is located within the apicoplast [12] ( Fig. 7b , top panel). Deletion of PDH in the rodent malaria parasite P. yoelii results in a defect in the parasite’s ability to mature during the late liver stage, and the parasites cannot initiate a blood stage infection [15] . However, the parasites are able to undergo a normal intraerythrocytic cycle, suggesting that PDH is not essential for intraerythrocytic growth of the parasite [15] . A finding that appears to be supported by the suggestion that the only essential apicoplast metabolic pathway is isoprenoid precursor biosynthesis [33] . Our observation that 3D7-PDH + parasites are resistant to oxythiamine in thiamine-free medium is consistent with Pf PDH being a target of oxythiamine and with the enzyme being essential for intraerythrocytic parasite growth. A similar argument can be made for Pf OxoDH. In eukaryotes, Pf OxoDH is a mitochondrial protein and we confirm that this is also the case in P. falciparum ( Fig. 7b , bottom panel). Pf OxoDH catalyses the synthesis of succinyl-CoA from 2-oxoglutarate ( Fig. 8 ). In P. falciparum , succinyl-CoA is required (in the first step) for the de novo haem synthesis, which is believed to be an essential pathway for the parasite [34] . One interpretation of our data, therefore, is that both Pf OxoDH and Pf PDH (both of which we show bind to OxPP generated from oxythiamine) are essential for intraerythrocytic parasite proliferation. Overexpression of just one of the two enzymes overcomes OxPP-induced inhibition of the other by acting as an OxPP sink, and thereby reducing the effective concentration of toxic OxPP within the parasite ( Fig. 4 ). We cannot, however, exclude the possibility that neither (or only one) of them is essential for intraerythrocytic parasite development. Overexpression of Pf PDH or Pf OxoDH could simply serve to steer OxPP away from an additional TPP-dependent enzymes—the real targets of oxythiamine’s antiplasmodial activity. In fact, the antiplasmodial activity of oxythiamine is likely to involve the simultaneous inhibition of multiple essential TPP-dependent enzymes. Our demonstration that heterologously expressed Pf PDH E1 and Pf OxoDH E1 are both capable of accepting 2-oxoglutarate and pyruvate as substrates ( Table 1 ) also opens up the possibility that both enzymes are capable of compensating for the functionality of the inhibited enzyme. Whether this would be possible, given the apparent distinct localization of Pf OxoDH and Pf PDH ( Fig. 7b ), remains to be seen. For this compensatory functionality to take place, it would require that the substrates (2-oxoglutarate and pyruvate) for each enzyme have access to both enzymes in their respective organelles. Their reaction products (succinyl-CoA and acetyl-CoA) would also need to be able to leave the surrogate organelle in which they were synthesized and, if necessary, enter the organelle within which they are required ( Fig. 8 ). The movement of these substrates and products across the mitochondrial and apicoplast membranes would be expected to take place via specific transporters. Another possibility, however, is direct exchange of metabolites between the mitochondrion and apicoplast ( Fig. 8 ). These organelles are known to be in very close proximity of each other [35] , [36] , [37] , presumably because of the shared biosynthetic pathways (for example, haem biosynthesis [4] , [38] ), and direct metabolite exchange might therefore be possible. In summary, our data validate thiamine utilization by P. falciparum as an antimalarial drug target. In addition, given that both the apicoplast and the mitochondrion have been suggested to possess pathways that are viable antimalarial drug targets [39] , [40] , [41] , [42] , the demonstration here that a single drug is shown to interact with enzymes in both of these organelles, and inhibit at least one pathway that is essential to the intraerythrocytic development of the parasite, provides support for a multi-target antimalarial strategy using a single pharmacophore, potentially delaying the development of resistance. Our data also provide novel insights into possible redundancies between the mitochondrial and apicoplast biochemical pathways. Materials Albumax II, HEPES and gentamycin, TRIZOL, Super-ScriptIII Reverse Transcriptase, SuperScript III One-Step RT-PCR System with Platinum Taq DNA Polymerase and RNaseOUT were obtained from Invitrogen. 2.5 RealMasterMix/20 × SYBR Green kit was purchased from 5 PRIME, Germany. Automated sequencing of nucleic acids was done by Seqlab, Germany. [ 3 H]Hypoxanthine (specific activity 30 Ci mmol −1 ; 0.03 mM) was purchased from American Radiolabeled Chemicals, and Microscint-O scintillation fluid was from PerkinElmer. Restriction enzymes and ligase were purchased from New England Biolabs, USA. Oligonucleotides were from Sigma-Aldrich, Germany. The cloning vector pASK-IBA3, Strep-Tactin-Sepharose, monoclonal Strep-tag II antibody, anhydrotetracycline and desthiobiotin were from Institut für Bioanalytik (IBA, Germany). The DNaseI was purchased from Promega, Germany, the vac SVC100 was purchased from Savant, Germany, and the Diode Array Detector was purchased from Dionex, USA. [U- 14 C] ATP (50 Ci mmol −1 ) was from ARC, USA. PEI-cellulose F-coated Polygram sheets were from MERCK, Germany. All other chemical reagents were purchased from Sigma-Aldrich. Buffy coat-poor group O + erythrocytes were provided by the Canberra Branch of The Australian Red Cross Blood Service, and A + erythrocytes were purchased from the Blood Bank of University Medical Center Hamburg-Eppendorf, Germany. RPMI-1640 culture medium with bicarbonate was obtained from the John Curtin School of Medical Research Media Facility (Australia) and AppliChem (Germany). ‘Complete medium’ was prepared by supplementing the RPMI-1640 culture medium with 25 mM HEPES, 11 mM D-glucose, 200 μM hypoxanthine, 24 μg ml −1 gentamycin and 0.6% (w/v) Albumax II. ‘Thiamine-free medium’ was prepared according to Sigma-Aldrich’s RPMI-1640 culture medium formulation except that thiamine was omitted. ‘Low-hypoxanthine medium’ (either in the presence or absence of thiamine) was prepared by supplementing RPMI-1640 culture medium with 25 mM HEPES, 11 mM D-glucose, 3 μM hypoxanthine, 24 μg ml −1 gentamycin and 0.6% (w/v) Albumax II. A medium with a high thiamine concentration was prepared by supplementing the ‘thiamine-free medium’ with 296 μM thiamine. In vitro culture of P. falciparum Intraerythrocytic 3D7 and transgenic (see below) strains of P. falciparum parasites were maintained in continuous culture as described previously [43] with modifications [44] , [45] . Heterologous expression of Pf PDH E1 and Pf OxoDH E1 The open-reading frames encoding either OxoDH E1 or PDH E1 (α and β) were amplified from P. falciparum 3D7 total RNA using the SuperScript III One-Step RT-PCR System with Platinum Taq DNA Polymerase and the oligonucleotides shown in Supplementary Table S1 . The PCR products obtained were digested with either Bsa I only or Sac II and Nco I and cloned into the expression plasmid pASK-IBA3, yielding the expression constructs IBA3-OxoDH E1-strep, IBA3-PDH E1α-strep and IBA3-PDH E1β-his, respectively. Recombinant expression in Escherichia coli BLR (DE3) and PDH E1β-his co-purification were carried out as described previously [46] . Generation of transgenic parasite lines The transfection constructs were generated by PCR using Pfu-polymerase on the IBA3-OxoDH E1-strep, IBA3-PDH E1α-strep and Pf TPK-IBA3 (ref. 8 ) as templates using the oligonucleotides listed in Supplementary Table S1 . The resulting PCR products were digested with Kpn I, or Xma I and Avr II, and cloned into the transfection vector pARL1a [47] , yielding the respective constructs for overexpression pARL-OxoDH E1-strep, pARL-PDH E1α-strep and pARL-TPK-strep. The GFP chimeras pARL-OxoDH-E1-GFP and IBA3-PDH E1α-GFP contain the first 100 amino acids of the N terminus of the respective protein fused to GFP. The constructs and the pARL1a vector (as mock plasmid) were transfected into P. falciparum and selected as described previously [29] , [48] . Western blot and localization of transgenic parasites Transgenic parasites were identified by plasmid rescue (data not shown), and expression of the fusion proteins in the parasite was analysed by western blot using cell lysate and either a monoclonal anti-strep antibody (1:5000) or a monoclonal anti-GFP antibody (1:5000), and a secondary anti-mouse HRP coupled antibody (1:20000) as described previously [48] . GFP fluorescence of parasites, treated with 50 nM WR99210, was analysed by fluorescence microscopy, and counterstaining was performed using Hoechst 33342 (ref. 48 ) for nucleus and 0.833nM MitoTracker Red CMX-ROS to identify the mitochondrion. RNA extraction and reverse-transcriptase quantitative PCR Total RNA was extracted from asynchronous, saponin-isolated, transgenic parasites using TRIZOL following the manufacturer’s instructions, digested with RQ1-RNasefree DNaseI for at least 1 h at 37 °C, stopped by incubation for 10 min at 65 °C and extracted by isopropanol. Synthesis of cDNA was accomplished with 200 U Super-ScriptIII Reverse Transcriptase from 1 μg RNA using 0.5 mM dNTP, Random Primer (250 μg), 5 mM dithiothreitol and 40 U RNaseOUT in 20 μl for 2 h at 42 °C. Super-ScriptIII Reverse Transcriptase was omitted as negative control for the subsequent real-time quantitative PCR using 2.5 RealMasterMix/20 × SYBR Green kit as previously described [49] with the gene-specific primers (10 pmol each), designed with Primer 3 (ref. 50 ) yielding products of 80–90 bp ( Supplementary Table S2 ), and 50 ng cDNA prepared on the day of the experiment with the following amplification conditions: 95 °C for 2 min, followed by 35 cycles at 95 °C for 15 s, 49 °C for 20 s and 68 °C for 20 s, and a melting step ramping from 67–95 °C. In each experiment from separate preparations of cDNA, each sample was analysed in duplicate. Aldolase was used for normalization [51] . RNA extracted from the MOCK-plasmid-carrying parasite line served as calibrator, and relative changes in the target cell line were measured using the 2 −ΔΔCT method [52] . Analysis was performed with the Corbett Rotor-Gene 6.1.81 software. Specificity of amplification was ascertained by melting-curve analysis of each PCR product using 3D7 gDNA. Pulldown of strep-tagged Pf OxoDH E1 and Pf PDH E1 Parasites overexpressing Pf OxoDH E1-strep or Pf PDH E1-α-strep were separated from noninfected erythrocytes via a discontinuous Percoll-alanine gradient as described previously [53] , cultivated for 5 h at 37 °C in either thiamine-free RPMI-1640 medium containing 11 μM oxythiamine or thiamine-replete RPMI-1640 (containing 2.96 μM thiamine) in the presence or absence of 5.2 mM oxythiamine. The cells were washed in prewarmed (37 °C) human tonicity-PBS (1 min at 16 000 g ). The cell pellets, isolated from 300 ml culture and at least 10% parasitemia, were resuspended in 500 μl buffer W (100 mM Tris-HCl and 150 mM NaCl), subjected to three freeze-thaw cycles and sonified in a Branson sonifier at low input for 20 × 20s pulses before the soluble protein fraction was separated by a centrifugation step of 20,000 g for 2 h at 4 °C. Pf OxoDH E1-strep and PfPDH E1-α-strep were purified via affinity chromatography using 50 μl of packed streptactin-matrix. The samples were washed three times with buffer W, eluted with buffer W containing desthiobiotin and dried in the speed vac SVC100 before HPLC analysis. HPLC and MS analysis Commercially available thiamine, TPP and oxythiamine were used as HPLC standards (dissolved in water at a concentration of 100 μM). OxPP is not commercially available and was therefore synthesized enzymatically. Heterologously expressed and purified Pf TPK (15 μg), prepared as described previously [8] , was used to pyrophosphorylate 50 nmol of oxythiamine. The reaction, described previously [54] , was performed for 6 h at 37 °C, and the reaction products were subsequently dried in a speed vac SVC100. In a separate assay, the conversion of ATP to ADP in the presence of thiamine and [ 14 C]-labelled ATP was used to ensure a positive enzyme reaction. The identity of OxPP was confirmed using mass spectrometry. Mass spectra were recorded on an Agilent 6550 QTOF with attached Agilent 1260 Auto-sampler, Column Compartment and 1290 Binary Pump. Chromatographic separation was carried out using isocratic elution in an Agilent XDB-C18 RRHD column (1.8 μm, 2.1 × 100 mM) using a mobile phase of 95% 10 mM ammonium carbonate/5% acetonitrile. Calculated 426.0290 for C 12 H 18 N 3 O 8 P 2 S; found 426.0294 (0.98 p.p.m. difference). MS/MS fragmentation provided additional evidence that the peak at 426.0294 m / z is OxPP ( Supplementary Fig. S3 ). HPLC samples were analysed using a Dionex Ultimate 3000 RSLC HPLC system equipped with a Diode Array Detector set to 265 nm. The absorbance maxima for the standards were determined in preliminary experiments using 3D-FIELD with a range of 200–800 nm. A Phenomenex Kinetex C18 column (1.7 μm, 2.1 × 100 mM) with the appropriate guard column was used at 35 °C with a flow rate of 0.5 ml min −1 . The mobile phase consisted of 100 mM ammonium acetate, pH 7.0, containing 5% (v/v) acetonitrile. An injection volume of 5 μl was used. Enzyme assays Before determining the specific activity of the recombinantly expressed subunits of Pf PDH E1 (α+β, co-purified) as well as Pf OxoDH E1, their purity was verified by SDS-PAGE (data not shown). The enzyme activity was followed by photospectroscopy at 600 nm using the electron acceptor 2,6-dichloroindophenol sodium salt (DCIP) as described previously [55] . The reaction buffer (50 mM KH 2 PO 4 and 2 mM MgCl 2 , pH 7) contained 200 μM TPP, 80 μM DCIP, 2 mM pyruvate/oxoglutarate and 50 μg enzyme. Specific activity was calculated using the molar extinction coefficient of 21 mM −1 cm −1 of DCIP. The pyrophosphorylation of oxythiamine was determined by thin layer chromatography using [ 14 C]ATP as described previously [54] . The apparent K M value was calculated from rectangular hyperbola fitted curves using SigmaPlot computer software. In vitro antiplasmodial assay The in vitro antiplasmodial activity of oxythiamine was measured using the [ 3 H]hypoxanthine incorporation assay as described previously [45] , [56] , [57] . Infected erythrocytes were exposed to twofold serial dilutions of oxythiamine in the appropriate thiamine-free or thiamine-replete medium, containing low hypoxanthine (3 μM) in the 96-h assay. After freeze thawing, the cell lysates were collected onto glass fibre filters, immersed in scintillation fluid and the radioactivity counted using a 96-well plate scintillation counter. The data were fitted to sigmoidal curves using SigmaPlot software to estimate IC 50 values. In vivo antimalarial assay In vivo activity of oxythiamine was determined using methodology described previously [56] . Balb/c mice (females, 18–21 g, 8 weeks old) were obtained from the Animal Resources Centre, Canning Vale, Western Australia. Approval for the study was obtained from the Animal Ethics Committee, The Australian National University (protocol number F.BMB.31.07). Blood was collected from a donor mouse, diluted with saline to 5 × 10 7 P. vinckei vinckei -parasitized erythrocytes per ml and 200 μl injected intraperitoneally to infect each mouse to be used in the experiment. Two hours following infection, the animals were randomly selected and divided into two groups of seven or eight mice each and were orally administered by gavage with 400 mg kg −1 per day of oxythiamine or an equivalent volume of distilled water (negative control group). The drug was given once daily for 3 consecutive days (day 0–day 2). A small drop of tail blood was taken from each mouse on day 5 post infection/start of drug treatment for preparation of methanol-fixed and Giemsa-stained smears. The parasitemia was determined for each mouse by counting the number of parasitized erythrocytes in random fields of more than 1,000 erythrocytes. The parasitemia of each mouse was monitored daily, and mice with parasitemia >25% were euthanized. Parasite growth inhibition was determined by comparing the parasitemia of mice receiving the test compounds with those in the negative control group. Changes in the physical activity and body weight of mice were also monitored daily from the start of drug treatment for signs of toxicity, and the mean survival time for each group was evaluated. How to cite this article : Chan X. W. A. et al . Chemical and genetic validation of thiamine utilization as an antimalarial drug target. Nat. Commun. 4:2060 doi: 10.1038/ncomms3060 (2013).